Phase nucleation in curved space Nucleation and growth is the dominant relaxation mechanism driving first-order phase transitions. In two-dimensional flat systems, nucleation has been applied to a wide range of problems in physics, chemistry and biology. Here we study nucleation and growth of two-dimensional phases lying on curved surfaces and show that curvature modifies both critical sizes of nuclei and paths towards the equilibrium phase. In curved space, nucleation and growth becomes inherently inhomogeneous and critical nuclei form faster on regions of positive Gaussian curvature. Substrates of varying shape display complex energy landscapes with several geometry-induced local minima, where initially propagating nuclei become stabilized and trapped by the underlying curvature. In its classical picture, nucleation and growth (NG) starts with local fluctuations of an initial metastable phase leading to the formation of a small nucleus of the equilibrium phase [1] , [2] , [3] , [4] . Such nucleus involves local changes in the free energy of the system. On one hand, the formation of a nucleus of the less-energetic phase produces a decrease in the total free-energy scaling with its volume. On the other hand, it raises the energy by an amount that scales with the area of the interface separating the two phases. In the case of flat two-dimensional (2D) systems, the variation in the free energy due to the formation of a nucleus of radius R takes the expression [1] , [2] , [3] , [4] : where σ represents the surface tension and Δ f the difference in the local free energies of initial and final phases driving the phase transition. The competition of surface and volume terms produces the activated dynamics of NG. Only those fluctuating nuclei whose size overpass the critical value R c = σ /Δ f will propagate. All other nuclei collapse due to surface energy. On the other hand, phases lying on curved backgrounds [5] , [6] , [7] , [8] , [9] , [10] are not only commonly found in nature in systems like viral capsids, pollen grains, radiolaria and others but also they can be obtained in the laboratory in the form of soft crystal or liquid crystal phases by using colloidal particles [11] , [12] , [13] , [14] , block copolymers [15] , [16] , [17] , [18] , [19] , liquid crystals [20] , [21] , [22] , [23] and other self-assembled systems. Examples of phase nucleation on curved geometries in hard-condensed matter may include, among others, graphene [24] , [25] , epitaxial growth of helium [26] and Wigner crystals on rough surfaces [27] . In equilibrium, these phases display regular structures strongly coupled to the underlying geometry that are not only ideal model systems to study the interplay between order and curvature but also potential platforms for technological applications such as soft lithography [15] , [19] or defect functionalization [28] . Although experiments and theoretical calculations have contributed to unveil equilibrium configurations and energetics of topological defects in curved space, dynamical processes like crystallization and melting still remain marginally explored [29] , [30] , [31] , [32] . In this work, we obtain generic features of NG in 2D systems lying on arbitrary curved backgrounds. Our model is based on a Ginzburg–Landau free energy functional, which is sufficiently general, that can be applied to various physical systems and substrate’s geometries. For nearly-flat surfaces and geometries of constant curvature, we obtain all the relevant information related to NG in a closed analytical form. On more complex surfaces of varying curvature, we explore the effects of the underlying geometry on NG by using simulations. We show that in general, the free-energy barrier needed to form a critical nuclei is strongly dependent on the underlying curvature, being smaller (larger) for region of positive (negative) curvature. As a consequence, in geometries of varying curvature NG is an inhomogeneous process, first starting in regions of positive curvature. Also, due to the competing effects of positive and negative curvature, geometries of varying curvature are shown to display complex relaxation in free-energy landscapes, with several barriers and local minima, where initially propagating nuclei become stabilized and trapped by the underlying curvature. Additional effects coming from system’s thickness and strain contributions during crystallization are also considered and discussed in view of recent experimental work. Model Here we present a model to study how the underlying geometry affects the laws of NG in curved space. In general, the geometry of an oriented surface (that is, separating an ‘internal region’ from an ‘external region’ of three-dimensional (3D) space) can be completely characterized by the principal curvature maps κ i ( r )=±1/ R i ( i =1, 2), where R 1 ( R 2 ) is the radius of the smallest (largest) circle tangent to the surface at r , and the sign is positive (negative) if the circle is contained in the internal (external) region. Alternatively one can use the Gaussian K ( r )= κ 1 ( r ) κ 2 ( r ) and mean H ( r )=( κ 1 ( r )+ κ 2 ( r ))/2 curvature [33] . The case K =0 and H ≠0 represents a plane bent in only one direction. Since this surface can be flattened preserving the areas (Minding’s theorem [33] ), nucleation can be mapped to the case of a planar surface and thus results to be trivial. Non-trivial cases have non-zero Gaussian curvature but may have zero mean curvature as in the case κ 1 =− κ 2 , which represents a saddle. This clearly cannot be flattened preserving the areas and thus nucleation has to be revisited. In other words, the Gaussian represents an ‘intrinsic’ curvature and, as we shall see, results to be most important in describing physical processes on the surface. Below we show how the Gaussian curvature influences NG in curved geometries. The mean curvature is not only related with the geometry of the surface, but also it is tied to the definition of ‘internal’ and ‘external’ regions. For example, while crest have positive mean curvature and valleys have negative mean curvature, these values can be inverted by exchanging the definition of ‘internal’ and ‘external’ regions [33] . As we will see later, mean curvature will modify NG for 2D systems with thickness. We study the dynamics of first-order phase transitions through a scalar and real order parameter . Points on the surface are specified by a system of curvilinear coordinates r =( x 1 , x 2 ). In these coordinates, an infinitesimal arc length d s is given in Einstein notation by d s 2 ≡|d r | 2 = g αβ d x α d x β , where g αβ is the metric tensor. Depending on the physical system considered, the order parameter is or is not a conserved quantity [34] . For example, while conserved order parameters are required to study nucleation of binary mixtures or solid solutions, non-conserved order parameters are commonly used in studies of the liquid-to-crystal transition or in magnetic and spin-related phases. In general, the free energy of a mixed state in a system lying on a curved surface can be expanded in terms of the order parameter: where k B is the Boltzman’s constant, T the temperature and g is the determinant of the metric tensor [33] . In a curved surface the differential of area is so the first term in the free energy represents the contribution from a local homogeneous situation, where is the local free-energy areal density of a phase with an order parameter . For a two-phase system this term takes the typical double-well form [36] , [37] , [38] , with two local minima corresponding to the initial and final phases, separated by a local free-energy barrier. This can be written phenomenologically as: where η and ɛ are constants. Here the local free-energy difference driving the phase transition, typically controlled by temperature, is given by Δ f = f (0)− f (1). Note that Δ f ≡ ɛ /4 is proportional to the degree of supercooling in the system. The second term of equation 2 is the curved-space generalization of the gradient square term that penalizes the formation of interfaces [1] , [2] . In this Ginzburg–Landau approach the dynamics of the phase transition can be studied through a relaxational equation of the form: where τ is a characteristic time scale (for simplicity here we take τ ≡1), , n ≡0,1 for non-conserved and conserved order parameters, respectively, and ) is the Laplace–Beltrami operator, which is the curved-space generalization of the Laplacian [29] , [30] . Note that a more complex evolution equation in needed for conserved order parameters. For simplicity we concentrate on the time evolution of non-conserved order parameters. However, most results related to NG on curved geometries can be applied to both [34] , [35] . Critical nuclei and growth and dissolution laws We start by analysing the fate of a nucleus resulting from a spontaneous fluctuation, whose time evolution follows equation (4). In the following we make use of geodesic polar coordinates, which are the curved-space generalization of the polar coordinates [33] . We start by locating an origin O in the centre of the nucleus ( Fig. 1 ). Then, a point P located on the surface is associated to coordinates ( r , θ ). The coordinate r is defined as the geodesic distance between P and the origin O. Closed lines of constant geodesic distance r 0 are called geodesic circles, and at any point are orthogonal to the geodesics starting at O. The coordinate θ of the point P is the angle that the geodesic connecting O and P makes with a reference geodesic starting in O. 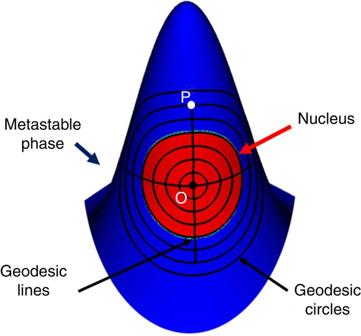Figure 1: Geodesic polar coordinates. In this work geodesic polar coordinates are used to describe the growth or collapse of a nucleus (red domain) in the sea of the metastable initial phase (blue). Here a point P on the surface has coordinates (r,θ), beingrthe geodesic distance to the origin O andθthe angle. Figure 1: Geodesic polar coordinates. In this work geodesic polar coordinates are used to describe the growth or collapse of a nucleus (red domain) in the sea of the metastable initial phase (blue). Here a point P on the surface has coordinates ( r , θ ), being r the geodesic distance to the origin O and θ the angle. Full size image In these coordinates the metric of any surface always take the simple form d s 2 =d r 2 + G ( r , θ ) dθ 2 , where the function G ( r , θ ) depends on the geometry of the surface through the equation , with K the Gaussian curvature of the surface, and G (0, θ )=0 (ref. 33 ). When using geodesic polar coordinates, the evolution equation (4) can be largely simplified to study steady-state solutions representing the growth or collapse of nuclei during NG. Here the evolution equation of a steadily propagating nucleus is decomposed (see Methods) in two equations for the interface profile (equation 5) and the propagation rate (equation 6). where the comoving coordinate X is given by X = r − R ( t ), R ( t ) is the radius of the nucleus at time t , a propagation constant, and the geodesic curvature is the local curvature of the geodesic circles providing information about the underlying geometry. It is interesting to note that for any geometry, the equation for the interface profile is always the same when written in geodesic polar coordinates. Its solution is exactly the same as found by Chan for NG on a plane [36] , [37] , [38] : . By contrast, equation (6) shows that the evolution of nuclei’s sizes is influenced by the underlying geometry through the geodesic curvature κ g . Note that for a planar geometry κ g ( R )≡1/ R gives the classical growth rate for NG on a plane. Although in the general case this is a complicated nonlinear ordinary differential equation, it can be solved in closed form for simple geometries, as shown below. In general, a nucleus will grow only if its initial radius R 0 exceeds the critical value R c , obtained by setting , that is: where represents the critical size for NG on a planar substrate, under the same external conditions. Thus, equation (7) shows that on a curved substrate, the critical radius will in general depend on both curvature (through κ g ) and supercooling (through ). A characteristic length associated to the curvature can be defined by . We can expect different regimes of NG depending on how large the ratio is. In the following sections we use equations (4), (6) and (7) to analyse how the geometry modifies NG on substrates with different distributions of curvature. Nucleation on nearly-flat substrates For cases when the critical nucleus is very small as compared with curvature , equally valid for NG far from the coexistence line or for slightly curved geometries, the geodesic curvature can be approximated through a series expansion of the form where K 0 is the Gaussian curvature of the substrate evaluated at the centre of the nucleus. Using this expansion in combination with the equation for the critical nuclei (equation 7), we get a critical radius that can be written in the form: where Γ K is a geometric factor given by: Thus, under same external conditions, the curvature modifies the process of NG and the critical nucleus will be smaller for regions of positive curvature, like crests and valleys ( K 0 >0), and larger for negative curved regions like saddles ( K 0 <0). The energy needed to form a small nucleus of radius r on the curved substrate can be written as Δ F ( r )=− A ( r )Δ f + P ( r ) σ , where and represent the area and perimeter of a geodesic circle with a first-order correction due to curvature. The height of the free-energy barrier for nucleation Δ F c is obtained by evaluating Δ F ( r ) at the critical size, and can also be written as: where is the energy barrier on a planar geometry. This last expression shows how (locally) the height of the barrier for nucleation is modified by the underlying geometry, decreasing (increasing) for regions of positive (negative) Gaussian curvature. The reason for this is simply geometrical. Given a small nucleus, the ratio between the perimeter and area enclosed is smaller for surfaces with positive curvature (and larger for negative curvature). Thus, for positive curvature, the contribution of the bulk term of the free energy is larger than the interfacial term, producing a smaller free-energy barrier for nucleation and a smaller critical size. Note that the last expression for the free-energy barrier for NG in a curved geometry resembles the classical result of heterogeneous nucleation and growth , where the free-energy barrier is modified by a function f ( θ ) of the wetting contact angle θ of the nuclei with the underlying substrate [1] , [2] . However, in classical heterogeneous nucleation, the critical size is not modified by the wetting angle θ . This is different from nucleation on curved space, where the underlying curvature affects both free-energy barriers and critical sizes. These results simply show that the underlying curvature can break the homogeneity of space, such that NG on a substrate of varying curvature becomes inherently inhomogeneous. In the following sections we consider NG for more general cases where the effects of the underlying geometry are much stronger . Nucleation on surfaces of constant curvature For spherical substrates, the Gaussian curvature is constant and positive K =1/ a 2 , with a the radius of the sphere. Here the geodesic curvature is simply written as κ g ( r )=1/[ a tan( r / a )], and the critical size for NG (equation 7) takes the form: Thus, the critical size monotonously decreases when decreasing the radius of the spherical substrate, meaning that for positive curvature NG is favoured for higher curvatures. The reason for this is again geometrical: on the surface of spheres, circles have more enclosed area for a given perimeter (as compared with the plane), and the ratio surface-perimeter increases when increasing the curvature. Given an initial nucleus of size R 0 , its temporal evolution is obtained through equation (6), which can be integrated in a closed form giving the implicit relation R = R ( t ): This is the growth ( R 0 > R c ) or dissolution law ( R 0 < R c ) for NG on spheres, and reduces to the classical result obtained by Chan for NG on a flat plane [36] , [37] , [38] , when taking the Euclidean limit R c << a . To test the accuracy of these analytical predictions, here we developed numerical simulations of NG on spherical substrates (see Methods). 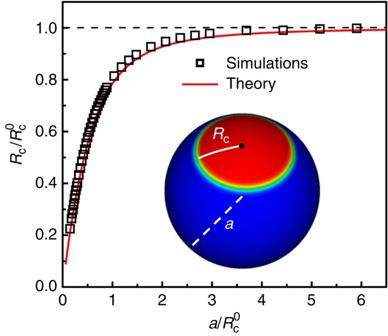Figure 2: Critical size for NG on spheres. The plot shows the critical (geodesic) radiusRcas a function of sphere radiusa, both quantities normalized with the critical size for nucleation on a plane, for simulations (symbols) and theoretical prediction (line). Note how the critical size decreases when increasing the curvature (a→0). As the underlying curvature decreases (a→∞) the critical size for NG converges to the value find for the flat plane. Figure 2 shows the excellent comparison between the theoretical prediction equation (11) (line) and simulations (symbols) for the critical size R c as a function of the radius a of the spherical substrate, normalized with the critical size on a plane . This plot clearly shows that nucleation is enhanced for high curvatures (smaller spheres). Note also that as the size of the sphere increases, the critical size for NG converges to the result obtained for the flat plane (vanishing curvature). Figure 2: Critical size for NG on spheres. The plot shows the critical (geodesic) radius R c as a function of sphere radius a , both quantities normalized with the critical size for nucleation on a plane , for simulations (symbols) and theoretical prediction (line). Note how the critical size decreases when increasing the curvature ( a →0). As the underlying curvature decreases ( a →∞) the critical size for NG converges to the value find for the flat plane . Full size image We can also consider NG on substrates with constant negative curvature K =−1/ a 2 , surfaces known as pseudospheres [33] , which at any point display the same local saddle structure. In this case the geodesic curvature is simply written as κ g ( r )=1/[ a tanh( r / a )], and the expression for the critical radius takes the form: Note that in general, all the expression for NG on pseudospheres are identical to the results obtained for spheres, when replacing the harmonic by hyperbolic functions. Contrary to spheres, here the critical size for NG monotonously increase when decreasing the radius a of the pseudosphere. 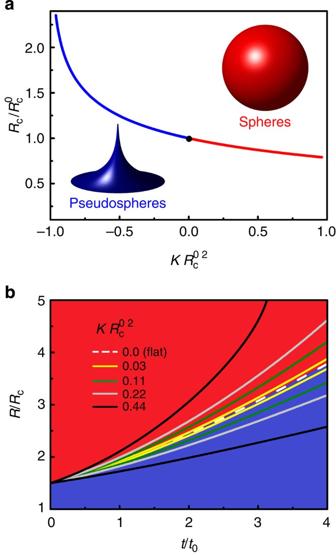Figure 3: NG in surfaces of constant curvature. (a) Critical size for nucleationRcas a function of Gaussian curvatureKfor substrates of constant Gaussian curvature, normalized with the critical size on a plane. The plot shows that the critical size for NG is larger for pseudospheres (K<0, blue line) as compared with spheres (K>0, red line) of the same curvature. Planar substrates (K=0), indicated with the black dot, have critical sizes between spheres and pseudospheres. (b) Time evolution of growing nucleiR(t) on substrates of positive (curves in the red region) and negative (curves in the blue region) constant curvature. HereRandtare normalized with the critical sizeRcandt0=Rc/v. Lines in the red (blue) zone represents the growth of nuclei in spheres (pseudospheres). Continuous lines of the same colour represent substrates on the same curvature (in absolute value), and the dashed line represents the growth law on a planar geometry. The growth of nuclei is faster (slower) for substrates of positive (negative) curvature. Note how the evolution converges to the growth law of NG on a plane as the curvature of spheres or pseudospheres decreases. Figure 3a shows a comparison for the critical size for nucleation on spheres and pseudospheres, where the critical radius R c is written as a function of the Gaussian curvature K of the substrate (this expression is valid for both positive and negative curvature). This plot represents a universal law of NG on substrates of constant curvature, generalizing the well-established results for NG on a plane. Here it is clear that the critical size for nucleation is bigger for pseudospheres as compared with spheres of the same curvature. Planar substrates, indicated with a black dot, have critical sizes between spheres and pseudospheres. Note also that Fig. 3a shows that the critical size for nucleation R c deviates from the result on a planar geometry for curvatures of the order , where for this substrates R K ≡ a , as expected. Figure 3: NG in surfaces of constant curvature. ( a ) Critical size for nucleation R c as a function of Gaussian curvature K for substrates of constant Gaussian curvature, normalized with the critical size on a plane . The plot shows that the critical size for NG is larger for pseudospheres ( K <0, blue line) as compared with spheres ( K >0, red line) of the same curvature. Planar substrates ( K =0), indicated with the black dot, have critical sizes between spheres and pseudospheres. ( b ) Time evolution of growing nuclei R ( t ) on substrates of positive (curves in the red region) and negative (curves in the blue region) constant curvature. Here R and t are normalized with the critical size R c and t 0 = R c / v . Lines in the red (blue) zone represents the growth of nuclei in spheres (pseudospheres). Continuous lines of the same colour represent substrates on the same curvature (in absolute value), and the dashed line represents the growth law on a planar geometry. The growth of nuclei is faster (slower) for substrates of positive (negative) curvature. Note how the evolution converges to the growth law of NG on a plane as the curvature of spheres or pseudospheres decreases. Full size image Figure 3b shows the time evolution of the size R ( t ) of growing nuclei on different substrates of positive (curves in the red region), null (dashed curve) and negative (curves in the blue region) constant curvature. This plot clearly shows that the growth of nuclei is faster (slower) for substrates of positive (negative) curvature, as compared with the plane. From the plot it is also clear how the evolution law converges to the law of NG on a plane, as curvature of spheres or pseudospheres decreases (dashed line). In what follows we consider NG on more complex geometries, where the varying curvature will produce richer free-energy landscapes and intricate relaxation paths towards equilibrium. Nucleation on surfaces of varying curvature In general, for substrates of non-constant curvature K , it can be difficult to obtain closed analytical expressions for the polar coordinates, needed to describe NG. In addition, for complicated geometries, we can expect the geodesic curvature to be not only function of the geodesic radius r but also of the polar angle θ , κ g = κ g ( r , θ ). In such cases the breaking of the radial symmetry makes the simplification of the evolution equation (4) much harder, and in general, other parameters related to shape in addition to size would be needed to describe the nuclei’s evolution. Given that the critical radius is strongly dependent on curvature ( Fig. 3a ), complicated geometries may induce complexities in the free-energy landscape for NG. Also, for substrates of varying curvature, we can expect that the opposite effects of positive and negative curvature will induce the acceleration or deceleration of interphases travelling through different regions ( Fig. 3b ), adding complexity to the relaxation paths towards the equilibrium phase. To unveil the dynamics of NG on more complex geometries, we developed numerical simulations (see Methods) for geometries in which the surface height at position ( x , y ) is given by Z = A cos(2 πx / L ) cos(2 πy / L ) (see the the surface in Fig. 4a–e ), where the curvature is symmetrically distributed into positive and negative curved regions. 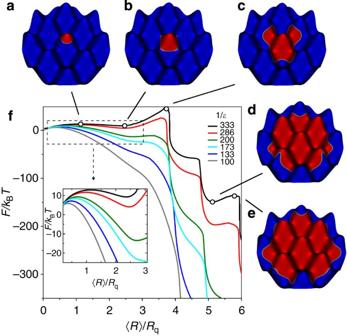Figure 4: NG in a sinusoidal geometry. (a–e) show snapshots of the simulation of growing nuclei seeded at a bump, which display characteristic features in the free-energy landscape for NG. (f) Free-energy barriers for NG on a fixed geometry and different degrees of supercoolings.Rqrepresents a measure of the roughness of the substrate. For high supercoolingsthe free energy display a single barrier. The inset shows the evolution of this barrier with the different supercoolings. The presence of negative curvature induces the formation of local minima an extra barrier for smaller supercoolings. Closer to coexistencea new minima and barrier appear as a consequence of the negative curvature of the next nearest saddles. Figure 4: NG in a sinusoidal geometry. ( a – e ) show snapshots of the simulation of growing nuclei seeded at a bump, which display characteristic features in the free-energy landscape for NG. ( f ) Free-energy barriers for NG on a fixed geometry and different degrees of supercoolings . R q represents a measure of the roughness of the substrate. For high supercoolings the free energy display a single barrier. The inset shows the evolution of this barrier with the different supercoolings. The presence of negative curvature induces the formation of local minima an extra barrier for smaller supercoolings . Closer to coexistence a new minima and barrier appear as a consequence of the negative curvature of the next nearest saddles. Full size image Figure 4f shows the free-energy landscape for nuclei initially seeded on the top of a bump (local positive curvature) for different degrees of supercooling . Here 〈 R 〉 acts as a collective coordinate and is defined as the geodesic distance between the interface and the centre of the seed averaged along the perimeter, and R q is the root mean squared distributions of heights, being a parameter representing the substrate’s roughness. Figure 4a–e shows shape and sizes of nuclei inducing distinctive points in the free-energy landscapes for NG. Figure 4f shows that for high supercoolings the system displays a single barrier for NG, as found for systems of constant curvature (plane, spheres or pseudospheres). The inset in Fig. 4f shows the expected enlargement of this barrier as the supercooling decrease. Remarkably, for low degrees of supercoolings, multiple barriers appear with local minima in between. Starting from low supercooling, a change of slope occurs around 〈 R 〉/ R q ∼ 2.5, which gives a local minima for . This 〈 R 〉 corresponds to the region in which the interface of the nuclei starts to approach the first neighbouring saddles (see Fig. 4b for a nucleus of this size). Clearly, this is a geometrical effect coming from an increase of surface energy of nuclei due to the approach to a negative curved region. Thus, initially propagating nuclei become equilibrated and trapped by the negative curvature of the saddles. The escape from these regions requires the overcoming of an extra barrier associated with a much larger critical size 〈 R 〉/ R q ∼ 3.5 ( Fig. 4c ). Here we note that for small supercooling on a periodically curved substrate it is possible to obtain a microemulsion state as a metastable thermodynamic phase. These geometries are such that practically all nucleation events will take place in regions of high positive curvature and the nuclei will be unable to invade regions of negative curvature. Thus, at low supercooling, the system will remain arrested in a metastable microemulsion state that share characteristics of both phases with interesting perspective for applications. The formation of emulsion phases are typical of systems with a conserved order parameter, like the familiar patterns obtained in oil–water mixtures [39] . These are non-equilibrium states that evolve in time according to a self-similar mechanism. However, on flat geometries, emulsions cannot be obtained for non-conserved order parameters, like crystallization, because once a nucleus overcomes the critical size it freely propagates throughout the system. As the coexistence line is approached, the critical nuclei grow in size, feeling the presence of other curved regions of the substrate. For a new local minimum arises for nuclei of sizes around 〈 R 〉/ R q ∼ 5. This minimum corresponds to the trapping of nuclei by the negative curvature of the next nearest saddle points ( Fig. 4d ), producing the formation of an extra barrier associated to a larger critical size 〈 R 〉/ R q ∼ 6. It is interesting to note here that this second geometry-induced barrier has a much lower height as compared with the previous. This is just a consequence of how the curvature is distributed on these sinusoidal substrates. For the second barrier, the negative curvature of the next nearest saddles is in part compensated by the positive curvature of the nearest positive-curved bumps, such that a lower activation is required to escape from these regions. Thus, close to coexistence, the energy landscape displays a ‘ratchet-like’ form, where the system relaxes by exploring subsequent metastable states of bigger size and smaller activation energy. 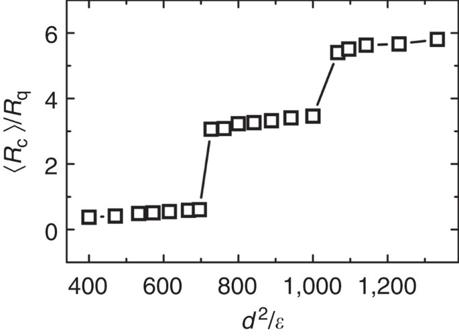Figure 5: Critical size for NG in a geometry of varying curvature. As a consequence the varying curvature in degree and sign, the critical sizeRcin sinusoidal geometries displays discontinuous jumps when plotting as a function of the supercooling. Thexaxis is normalized with. Figure 5 shows the evolution of the critical size R c for NG as a function of the degree of supercooling . As expected, the critical size decreases with supercooling. However, the formation of new minima and extra barriers as supercooling is varied, originate abrupt jumps in the critical size for nucleation. Figure 5: Critical size for NG in a geometry of varying curvature. As a consequence the varying curvature in degree and sign, the critical size R c in sinusoidal geometries displays discontinuous jumps when plotting as a function of the supercooling . The x axis is normalized with . Full size image Note that in complex geometries, it is also possible that the spatial location where the critical nuclei reside, could change as supercooling is varied, originating thus not only jumps in critical sizes but also sudden changes in the surface locations where critical nuclei develop. Effect of the mean curvature Up to now we have considered the effects of the Gaussian curvature K on NG. This is the only curvature that modifies the laws of NG in 2D systems of negligible thickness. Here we consider physical systems where the thickness δ of nuclei cannot be neglected, but where the NG process can still be considered as fundamentally 2D ( δ ≪ R c ). In such cases, a system with thickness can be modelled by two parallel surfaces displaced by [40] , [41] , where is the normal to the surface (see an scheme of the system in Fig. 6a ). As shown below, in such cases not only the Gaussian curvature K but also the mean curvature H plays an important role in NG. 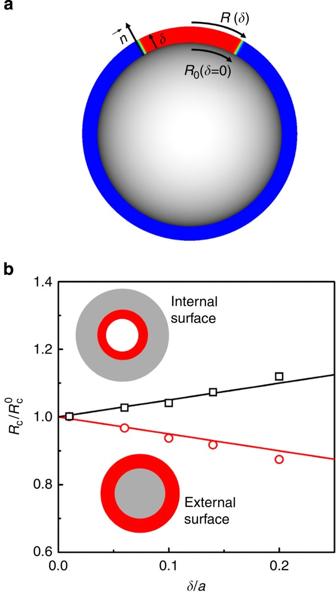Figure 6: NG in 2D systems with thickness. (a) Cartoon showing a scheme of a nucleus in a surface with normaland thicknessδ. Here while in the internal layer the nucleus has a radiusR0≡R(δ=0), on the external layer the nucleus has a bigger sizeR(δ)>R0. (b) Nucleation in spherical geometries of radiusafor systems with thicknessδ. The plot compares simulations (symbols) and theory (lines) for critical sizeRc(normalized with the critical size in a planar geometry) as a function of thicknessδ. The data on the bottom (top) corresponds to NG on external (internal) surfaces, whereRcdecreases (grows) withδ. Figure 6: NG in 2D systems with thickness. ( a ) Cartoon showing a scheme of a nucleus in a surface with normal and thickness δ . Here while in the internal layer the nucleus has a radius R 0 ≡ R ( δ =0), on the external layer the nucleus has a bigger size R ( δ )> R 0 . ( b ) Nucleation in spherical geometries of radius a for systems with thickness δ . The plot compares simulations (symbols) and theory (lines) for critical size R c (normalized with the critical size in a planar geometry ) as a function of thickness δ . The data on the bottom (top) corresponds to NG on external (internal) surfaces, where R c decreases (grows) with δ . Full size image The effects of finite thickness can be studied by considering the energy of formation of a nucleus: where the volume V and surface area A can be calculated by considering the nucleus as composed of different layers. On each of these layers the section of the nucleus is (approximately) a geodesic circle, but due to the presence of curvature, the radius of these circles will be in general, a function of the thickness. Then, the volume and area can obtained by integrating the area and perimeter of the geodesic circles in the thickness of the system (see Methods). In the limit of small thickness ( δ << R ) and small curvatures , the energy of formation of nuclei can be expanded leading to a simple expression for the critical size for NG (see Methods): where again Γ KH represents a geometric factor, but now this factor is a function of both curvatures and thickness: Thus, as previously found for the Gaussian curvature K 0 , in general, the presence of non-zero mean curvature H 0 and finite thickness δ will contribute to the formation of critical nuclei during NG. Note however that as the mean curvature is related to the way the surface is embedded in 3D Euclidean space, the critical size for NG will be very different if the process develops on the external or internal surface of the substrate. For example, for the case of cylindrical substrates, it will be much easier to nucleate in the external surface of the cylinder than on its internal face . A similar behaviour was previously observed by using Monte Carlo simulations of NG dynamics in colloidal suspensions [42] . Figure 6b shows the good agreement between the theoretical expression equation (15) and numerical simulations for NG on spheres for nuclei of different thickness δ . Note how the critical size decrease with δ for NG on the external surface of the sphere, but increase with δ on an internal surface. Effect of elastic frustration In general, when a crystal is forced to reside on a curved surface, some lattice bonds necessarily compress or stretch, giving rise to an increase of the strain energy, geometrically frustrating the formation of crystal bonds [5] , [6] , [7] , [8] , [9] . In some cases, such elastic distortions can be released by introducing topological defects in the lattice on particular regions of the substrate. In a recent experiment, the effects of this elastic frustration on NG has been explored by following the dynamics of 2D growing colloidal crystals on spherical substrates [32] . Here the colloidal particles were constrained to reside on the curved interface of water droplets dispersed in oil. This study revealed the presence of an elastic instability as a main consequence of the high geometric frustration in the crystallites. Due to the rapid increase of the strain energy with size, the nuclei tend to grow in ramified fractal-like form on spheres rather than in the typical compact structure observed in planar geometries. The effects of curvature and frustration on crystallization has also been recently studied in experiments of 3D heterogeneous nucleation on the surface of curved substrates [43] , [44] . Here foreign particles are located inside colloidal suspensions, acting as seeds for crystallization, giving rise to a heterogeneous nucleation process, which starts on the surface of a curved hard wall (the surface of the foreign particles) [45] . Such studies have also shown how curvature and geometric frustration can modify NG. It was found that although critical nuclei still form on the surface of the substrates, they tend to detach when growing, mainly because the curvature produce strains in the crystal lattices (some crystal’s bonds would need to stretch or compress in order to adjust to the surface geometry), which largely increases the elastic free energy of growing nuclei. Although such NG processes are mainly 3D, and then in principle different to the 2D processes considered here, some similarities are found. For example, due to the effects of mean curvature H 0 and thickness δ the NG is found to be different if the process develops on the outer or inner surface of the substrates. The effects of elastic frustration can be incorporated in our model by adding the corresponding elastic free energy to the functional in equation 2. In general, the elastic energy of a curved crystalline monolayer on a curved substrate can be written as: where Y is the Young modulus of the crystal and χ is the Airy stress function, which is dependent of both underlying curvature K and presence and location of topological defects in the crystal. In the case of spherical substrates of radius a , and for small nuclei of size R containing no defects, the elastic free energy results in (ref. 32 ). 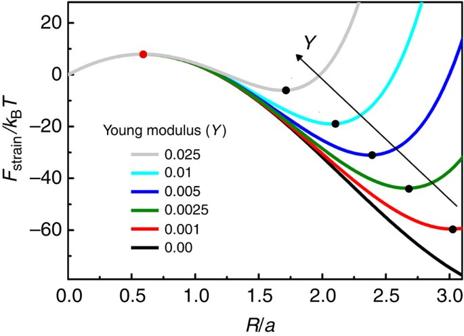Figure 7: NG in a spherical substrate under elastic frustration. The plot shows the energy landscapeFfor NG for different Young modulusY, whereRis the nuclei’s geodesic radius andathe sphere radius. For crystal patches having no defects, the free energy displays an absolute minima related to the formation of nuclei reaching equilibrium sizes (black dots) in addition to the conventional thermal barrier (red dot). Figure 7 shows free-energy barriers for NG on spherical substrates, for defect-free crystal nuclei of different Young modulus. Here in addition to the thermal barrier (red dot), the fast increase in the strain of the nuclei with R produces an absolute minimum in the energy landscape (black dots), such that a growing nuclei would reach an equilibrium size, being unable to propagate throughout the system. One way to escape from this energy minimum is by distorting the nuclei shape in less-compact structures, as observed in the experiments of Meng et al . [32] Figure 7: NG in a spherical substrate under elastic frustration. The plot shows the energy landscape F for NG for different Young modulus Y , where R is the nuclei’s geodesic radius and a the sphere radius. For crystal patches having no defects, the free energy displays an absolute minima related to the formation of nuclei reaching equilibrium sizes (black dots) in addition to the conventional thermal barrier (red dot). Full size image Note that for cases where the lattice structure is very soft (where topological defects have low core energies), it is conceivable that the system would rapidly relax the strain energy through the formation of topological defects. In such cases, we can expect that the strain-free energy contribution do not play a major role in the nucleation dynamics and therefore we can expect similar results for NG on curved geometries as in previous sections. In this work we have studied NG on curved geometries in systems where the imbalance of volume and surface free energies of nuclei directs the phase transition. It is precisely the change of this imbalance with supercooling and local curvature that makes NG a rich and complex phenomena in curved space. In general, the critical size and propagation rate of nuclei are both strongly dependent on the underlying geometry. For large curvatures, the critical sizes can be severely modified ( Fig. 3a ). For example, for cases where the radius of curvature of the substrate is of the order of the critical size for nucleation on the plane , the critical size for nucleation is reduced in 35% for positive underlying curvature. Note, however, that for the same thermodynamic conditions the critical size becomes about 250% larger for negative underlying curvature. Because of this effect, substrates of varying curvature impose complex relaxation paths for NG, with several geometry-induced local minima, with interesting applications for phases deposited on substrates of controlled roughness. In general, the characteristic time τ m that a system spends in a given metastable state roughly scales with its activation energy: (refs 1 , 2 ). Contrary to NG of two-phase systems in planar geometries, here the different local free-energy minima originated by the varying curvature would give rise to a full spectrum of relaxation times. Such spectrum, having the main information of how the relaxation process is developed, is a fingerprint of the way the curvature is distributed throughout the substrate. Due to the generality and simplicity of our model, we expect that the results obtained here could be applied to a variety of systems in condensed matter, and other fields concerned with the development of a new phase on a curved surface. Experiments of colloidal crystallization on curved surfaces could be carried out on capillary bridges of negative Gaussian curvature and null mean curvature, used in the studies of 2D curved crystalline structures and defects in refs 13 , 14 . The combined effects of Gaussian K and mean H curvatures and thickness δ on NG could also be experimentally addressed by confining block copolymers, liquid crystals or similar systems into different geometries [16] , like corrugated substrates [15] , [19] , spherical shells [20] or toroidal droplets [23] . In all these systems we expect that the interplay between geometry and phase nucleation will lead novel pattern formation phenomena that can be controlled to design useful supramolecular and soft materials. Equations describing the steady propagation of nuclei After the functional derivation in equation (4), the evolution equation for a non-conserved order parameter takes the form: Upon using geodesic polar coordinates, the Laplace–Beltrami operator can be written as [46] : where is the local curvature of the geodesic circles. For general geometries the Laplace–Beltrami operator takes a complex form, being dependent on both coordinates ( r , θ ). However, for surfaces with radial symmetry respect to the origin O, the geodesic curvature is only a function of the geodesic distance κ g ≡ κ g ( r ). In such cases we expect the nuclei to have radial symmetry, such that the Laplace–Beltrami operator takes the much simplified form . We can now describe steady-state solutions representing the growth or collapse of nuclei during NG. Here the motion of a steadily propagating interface can be described through a single combined coordinate X = r − R ( t ), where R ( t ) is the radius of the nuclei at time t . We assume that the interface is narrow respect to the nuclei radius R . Then we can take κ g ( r )≡ κ g ( R ) and rewrite the evolution equation in the comoving coordinates X , as the system of coupled equations (6) and (7) in the Results section. Simulations The simulations of NG in curved space performed in this work were developed by seeding an initial (geodesic) circular nucleus of a prescribed initial radius R 0 on a particular region of the substrate, and studying the temporal evolution through the numerical resolution of equation (18). The initial circular nuclei were obtained, for any underlying geometry, through a fast marching algorithm [47] . Equation (18) can be accurately solved through a finite difference scheme, forward in time and centred in space and periodic boundary conditions [29] , [30] . In the case of systems with finite thickness, the simulations were performed by numerically solving equation (18) through finite elements, with periodic and null flux boundary conditions. For different geometries and degrees of supercoolings ɛ , the critical sizes R c were obtained by finding the smallest nuclei, which is able to grow in time. The free-energy landscapes for NG were obtained by inserting the order parameter distribution , of growing or collapsing nuclei of size R ( t ), in the free-energy functional equation (2). Critical size in systems with thickness Given a nucleus in a curved system with thickness, some general conclusions can be drawn in the limit of small width δ and small critical size R c . To get the volume V and area A associated to the formation during nucleation (equation 14), the nucleus is considered as having different layers, where in each layer the nucleus has a circular shape. Thus, the volume and area can be obtained by integrating the area and perimeter of the geodesic circles in the thickness of the system. Here the perimeter P δ and area A δ of these circles can be written in the approximate form [33] : where R ( δ ) and K ( δ ) are the radius and Gaussian curvature in the δ -layer, given by: Here R 0 , K 0 and H 0 represent the size of nuclei and the Gaussian and mean curvatures evaluated on the surface of the substrate (for δ ≡0). The above expression for the Gaussian curvature is a well-known result that relates the Gaussian curvature of a surface K with the Gaussian K 0 and mean H 0 curvatures of a parallel surface displaced by , with the normal to the surface [40] , [41] . In this approximation, the area and volume of the nucleus take the simple forms: The replacement of these expressions in the energy of formation of a nucleus with thickness (equation 14), straightforwardly leads to the expression of the critical size for NG (equation 15). How to cite this article: Gómez, L. R. et al . Phase nucleation in curved space. Nat. Commun . 6:6856 doi: 10.1038/ncomms7856 (2015).